Complexity of biological scaling suggests an absence of systematic trade-offs between sensory modalities inDrosophila 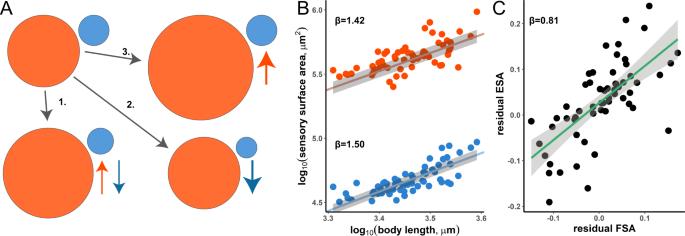Fig. 1: Analysing scaling relationships of eye and funiculus surface area [ESA (red) and FSA (blue)] reveals lack of inverse relationship between vision and olfaction in 59 species. AUsing ratios does not distinguish between a trade-off scenario (1.) from others where either vision (numerator) is strongly increased (2.) or olfaction (denominator) strongly decreased (3). Each scenario presented can result in the same EF ratio of 11.81 (the highest value in the dataset) when converted from a ratio of 5.54 (the lowest value in the dataset), where the circle area reflects the volume used to determine the EF ratio.BMCMC based phylogenetic regression models in BayesTraits V3.0.210of both surface areas reveals allometric scaling with body length. Indicated is the slope of each regression line based on phylogenetically controlled regressions, with confidence intervals as grey bands.CCalculating the residuals from B, performing a phylogenetic linear regression and plotting them reveals a positive relationship, i.e. an absence of an inverse relationship (confidence intervals as grey bands). Source data are provided as a Source Data file. 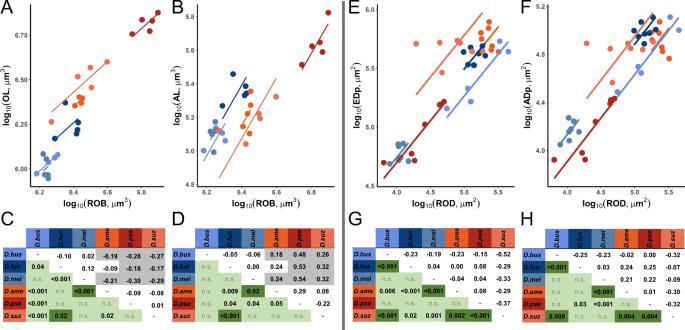Fig. 2: Analysing scaling relationships of vision and olfaction related structures in the brain and eye-antennal imaginal discs reveals a lack of inverse relationships between vision and olfaction despite strong variation in scaling between sixDrosophilaspecies. (A–B,E–F) The top row displays a plot of the visual and olfactory portion against the relevant allometric control (Rest of Brain, RoB, or Rest of Disc, RoD). Regression lines were derived from a SMATR12analysis, where slope differences could not be detected. The analysis revealed intercept differences, after which a species pair-wise analysis was conducted. (C–D,G–H) This pair-wise analysis (based on theWaldstatistic) is displayed in the bottom row. The green diagonal displays the significance of pair-wise differences. If the pair showed significant differences in the visual and olfactory portion this is indicated by dark green. The off diagonal indicates the difference between the intercepts. Opposing signs of intercept differences betweenCandDorGandHcould indicate an inverse relationship between a specific species pair where one structure is traded off against another. Cases which fit this description and show a shift are indicated by a grey background (excluding pair-wise comparisons with minor (<0.1 units) differences). Abbreviations: OL: optic lobe, AL antennal lobe, ROB rest of brain, EDp eye disc portion, ADp antennal disc portion, ROD rest of disc, n.s. not significant;D.bus=D. busckii(N= 4 brains; N= 5 imaginal discs),D.fun=D. funebris(N= 5;N= 8), D.mel=D. melanogaster(N= 5;N= 7), D.ame=D. americana(N= 5;N= 7), D.pse=D. pseudotalamancana(N= 5;N= 7), D.suz=D. suzukii(N= 5;N= 7). Source data are provided as a Source Data file. We used MCMC based phylogenetic regression models in BayesTraits V3.0.2 [11] to analyse the head sensory structure dataset, and linear models available through R (version 4.1.1 [17] ) standard packages as well as species-specific slopes tests using the R package smatr [12] for the brain and imaginal disc datasets (see Supplementary Code 1 file). For more detail, please see the Supplementary Methods . Reporting summary Further information on research design is available in the Nature Research Reporting Summary linked to this article.